A megacomplex composed of both photosystem reaction centres in higher plants Throughout the history of oxygen evolution, two types of photosystem reaction centres (PSI and PSII) have worked in a coordinated manner. The oxygen evolving centre is an integral part of PSII, and extracts an electron from water. PSI accepts the electron, and accumulates reducing power. Traditionally, PSI and PSII are thought to be spatially dispersed. Here, we show that about half of PSIIs are physically connected to PSIs in Arabidopsis thaliana . In the PSI–PSII complex, excitation energy is transferred efficiently between the two closely interacting reaction centres. PSII diverts excitation energy to PSI when PSII becomes closed-state in the PSI–PSII complex. The formation of PSI–PSII complexes is regulated by light conditions. Quenching of excess energy by PSI might be one of the physiological functions of PSI–PSII complexes. In oxygenic photosynthetic organisms, two photosystem reaction centres (PSI and PSII) cooperate to split water [1] . The regulation of photosynthesis has been studied based on the idea that all photosystems exist separately in thylakoid membranes. However, recent reports have questioned this concept. A megacomplex consisting of PSII, PSI and phycobilisomes was identified in cyanobacteria, in which phycobilisomes supply excitation energy to both photosystems [2] . Although the distribution of the two reaction centres is inhomogeneous in higher plants, PSI and PSII still have a chance to directly interact. The two reaction centres coexist in a flexible nonappressed region [3] , [4] , and about half of PSIIs exist in stroma thylakoids and grana margins where PSIs also exist [5] . Recently, Järvi et al . [6] reported coexistence of PSI and PSII complexes together with light-harvesting complexes (LHCs) in large-pore blue-native polyacrylamide gel electrophoresis (PAGE) from Arabidopsis , suggesting possible interaction between the complexes. In this study, we combined large-pore clear-native PAGE (lpCN-PAGE) and time-resolved spectroscopy to examine whether PSI and PSII interact with each other in Arabidopsis thaliana . Here, we show that about half of PSIIs are physically connected to PSIs in Arabidopsis thaliana . In PSI–PSII complexes isolated by lpCN-PAGE, excitation energy is transferred efficiently between the two closely interacting reaction centres. PSII diverts excitation energy to PSI when PSII becomes closed-state in the PSI–PSII complex. It may help to protect PSII from excess energy, and keep a balance between two photosystems. The formation of PSI–PSII complexes is regulated by light conditions. Energy transfer from the PSII reaction center to PSI in leaves First, we examined whether PSI–PSII complexes existed in A. thaliana by delayed fluorescence analysis. Delayed fluorescence with a time constant of ~20 ns at −196 °C is derived from charge recombination in PSII [7] , [8] . PSI and LHCII by themselves did not show delayed fluorescence in this timescale at this temperature ( Supplementary Figs 1 and 2 ), consistent with previous reports [9] , [10] , [11] . Therefore, the delayed fluorescence spectrum reflects the excitation distribution after direct excitation of PSII [12] . If PSI–PSII complexes do not exist, PSII does not transfer excitation energy to PSI, and the excitation energy generated by the charge recombination at PSII is distributed only in PSII even though the two reaction centres exist in the same place. On the other hand, in the case that PSI–PSII complexes exist, the energy is also distributed to PSI. Therefore, delayed fluorescence should appear in the PSI wavelength region at −196 °C if PSI–PSII complexes exist [12] . 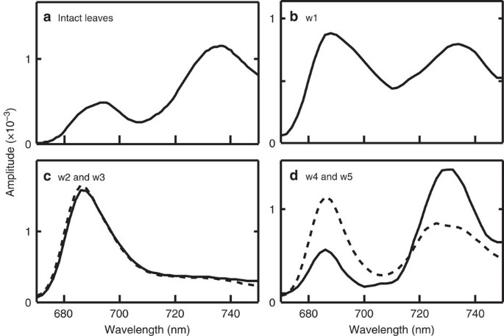Figure 1: Delayed fluorescence spectra obtained at −196 °C. Other lifetime components are shown inSupplementary Fig. 3. (a) Intact leaf of the wild type. (b–d) The w1–w5 samples from lpCN-PAGE gel pieces corresponding to the regions described inFig. 2. (b) The w1 sample. Decay curves were measured two times with a 1.2-ps interval and five times with a 24.4-ps interval. (c) The w2 (black solid line) and w3 (black dotted line) samples. Decay curves were measured two times with 1.2-ps and 24.4-ps intervals. (d) The w4 (black solid line) and w5 (black dotted line) samples. Decay curves were measured two times with 1.2-ps and 24.4-ps intervals. Excitation energy transfer from PSII to PSI was observed in the w1, w4 and w5 samples. Figure 1a shows the delayed fluorescence spectra of an intact leaf of the wild type measured at −196 °C. The delayed fluorescence spectrum showed a large peak in the PSI wavelength region (~735 nm) and a peak in the PSII wavelength region (~690 nm), indicating the existence of PSI–PSII complexes. After correction to remove the effects of differences in fluorescence quantum yield among chlorophyll forms ( Supplementary Fig. 3f ) [12] , we found that 48% of the excitation energy generated by charge recombination at PSII was transferred to PSI. Interestingly, this value was similar to the ratio of the relative distribution of PSII core proteins in unstacked regions (stroma thylakoids and grana margins) where PSI exists [5] . On the basis of the delayed fluorescence intensity, about 74% of PSI was calculated to be bound to PSII ( Supplementary Note 1 ). We also measured delayed fluorescence with a chlorophyll b -less mutant ( ch1-1 ), in which the LHCII level is drastically decreased, and five lhc mutants ( lhca1–4 and lhcb5 ) to check whether LHCs acted as linkers between PSI and PSII. All mutants showed a large PSI peak in their delayed fluorescence spectra ( Supplementary Fig. 4 , 6th lifetime component). These results suggested that LHCs were not required for PSI–PSII complex formation. Figure 1: Delayed fluorescence spectra obtained at −196 °C. Other lifetime components are shown in Supplementary Fig. 3 . ( a ) Intact leaf of the wild type. ( b – d ) The w1–w5 samples from lpCN-PAGE gel pieces corresponding to the regions described in Fig. 2 . ( b ) The w1 sample. Decay curves were measured two times with a 1.2-ps interval and five times with a 24.4-ps interval. ( c ) The w2 (black solid line) and w3 (black dotted line) samples. Decay curves were measured two times with 1.2-ps and 24.4-ps intervals. ( d ) The w4 (black solid line) and w5 (black dotted line) samples. Decay curves were measured two times with 1.2-ps and 24.4-ps intervals. Excitation energy transfer from PSII to PSI was observed in the w1, w4 and w5 samples. Full size image Isolation of PSI–PSII complexes by lpCN-PAGE Next, we isolated thylakoid membranes from the wild type, and separated the complexes by lpCN-PAGE. We observed that 26% of the excitation energy in PSII was transferred to PSI in the thylakoid membrane ( Supplementary Fig. 3e,f ). The detergent digitonin partially solubilized thylakoid membranes. The insoluble fraction contained ~60% of the chlorophyll and was composed of PSII–LHCII complexes; little PSI fluorescence was detected ( Supplementary Fig. 5 ). This indicated that the insoluble fraction was mainly composed of grana stack regions. The soluble fraction was subjected to large-pore gel electrophoresis. All soluble fractions passed through the stacking gel, indicating that the complexes were completely solubilized in the sample (also see Supplementary Fig. 6 ). The electrophoretic profile of the wild type was very similar to that in a previous report ( Fig. 2 ) [6] . The largest band was estimated as >2,400 kDa, and contained PSI, PSII, LHCII and LHCI revealed by silver staining, immunoblot analysis and liquid chromatography–mass spectrometry (LC–MS)/MS analysis ( Supplementary Figs 7–9 ) [6] , [13] . We called this green area the w1 sample. According to the estimate of protein amounts from LC–MS/MS data by the exponentially modified protein abundance index method, PSI, PSII, LHCII and LHCI subunits made up 94% in the w1 sample ( Supplementary Fig. 9 ). The second and third areas, referred to as w2 and w3 samples, respectively, were larger than 720 kDa ( Fig. 2 ), and assigned to PSII–LHCII complexes and comigrated PSI oligomers ( Supplementary Figs 7–10 ) [6] , [13] . In the range of 480–720 kDa ( Fig. 2 ), there was a broad green area that contained two distinct bands (thin broken arrows) and a faint broad green band (thin solid arrow). The heavier band was assigned to PSI–LHCI/II, and the lighter band was assigned to PSI–LHCI and comigrated PSII complexes [6] , [13] . lpCN/SDS–PAGE and immunoblot analyses revealed that the additional band indicated by the thin solid arrow in Fig. 2 contained both PSI and PSII ( Supplementary Figs 7 and 8a ). The lpCN-PAGE gel exhibited a green colour between the two distinct bands, indicating the presence of another complex(es) in this region. We divided this region into two samples, w4 and w5; the w4 sample contained the upper band and the faint broad band ( Fig. 2 ). 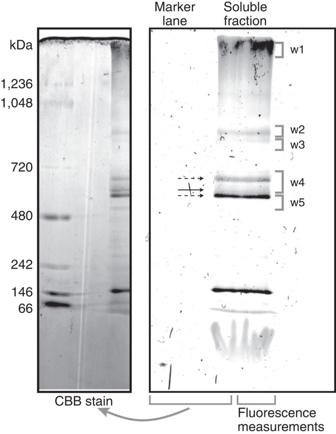Figure 2: lpCN-PAGE analysis of thylakoid membranes of the wild type solubilized by 1% digitonin. The marker lane and the left edge of sample lane were cut off and stained with Coomassie Brilliant Blue. The remaining sample lane was used for fluorescence measurements. Figure 2: lpCN-PAGE analysis of thylakoid membranes of the wild type solubilized by 1% digitonin. The marker lane and the left edge of sample lane were cut off and stained with Coomassie Brilliant Blue. The remaining sample lane was used for fluorescence measurements. Full size image Delayed fluorescence of isolated PSI–PSII complexes Then, we measured the delayed fluorescence spectra of these samples at −196 °C. In the w1 sample, the delayed fluorescence spectrum (18 ns) showed clear peaks in both the PSII and PSI wavelength regions, indicating excitation energy transfer from PSII to PSI ( Fig. 1b ). In the PSI wavelength region, the peak position was 735 nm, which was derived from low-energy chlorophylls in PSI–LHCI [14] , [15] . This result was consistent with the PAGE analysis and LC–MS/MS analysis ( Supplementary Figs 7–9 ), which showed the existence of a megacomplex composed of PSI, PSII, LHCI and LHCII in A. thaliana [6] . In the w1 sample, 26% of the excitation energy generated by charge recombination at PSII was transferred to PSI–LHCI at −196 °C ( Supplementary Fig. 3f ). Fluorescence originating from LHC antennae (~680 nm) decreased within 100 ps in the w1 sample ( Supplementary Fig. 3b , 1st component), indicating efficient energy transfer from LHCI and LHCII to the reaction centres. Hereafter, we call this megacomplex in the w1 sample the ‘larger PSI–PSII complex’. The w1 sample became more intense under milder solubilization, but the spectroscopic properties were not altered ( Supplementary Fig. 11 ). The delayed fluorescence spectra of the w2 and w3 samples ( Fig. 1c ) showed only a peak at 686 nm that was derived from PSII, despite the presence of a lot of PSI in these samples, reflecting a lack of energy transfer from PSII to PSI. This result clearly indicated that w2 and w3 did not contain PSI–PSII complexes. The delayed fluorescence spectra of the w4 and w5 samples showed clear peaks in both the PSII and PSI wavelength regions ( Fig. 1d ). These results indicated that w4 and w5 contained not only PSI–LHCI/II, PSI–LHCI and PSII dimers, but also a smaller PSI–PSII complex. At least 76% and 45% of the excitation energy generated by charge recombination at PSII was transferred to PSI in w4 and w5 at −196 °C, respectively ( Supplementary Fig. 3f ). The smaller PSI–PSII complex in w4 and w5 contained fewer LHCIIs ( Supplementary Figs 7–9 ). We assumed that the smaller PSI–PSII complex contained a PSI core and PSII monomer, while LHCII was bound to PSII and PSI peripherally in the larger PSI–PSII complex ( Supplementary Note 2 ; Supplementary Fig. 12 ). According to the blue-shifted PSI peak in the delayed fluorescence spectrum ( Fig. 1d ), some small subunits including Lhca might be lacking in the smaller PSI–PSII complex [16] , [17] . We found two types of PSI–PSII complexes, larger and smaller complexes. In the larger PSI–PSII complex, rapid energy migration and trapping occurred at room temperature. 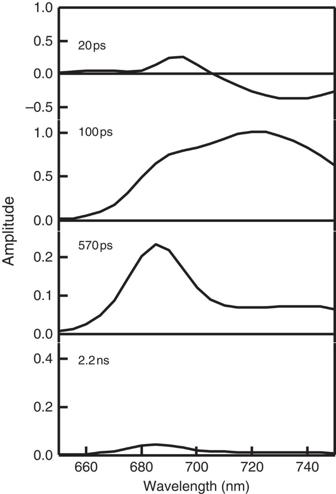Figure 3: Fluorescence decay-associated spectra of the w1 sample (20 °C). Decay curves were measured two times with a 2.4-ps interval. Lifetime components were normalized to the lifetime component of the largest amplitude in the sample. Figure 3 shows the fluorescence decay-associated spectra of the w1 sample (the larger PSI–PSII complex) at 20 °C. The 20-ps lifetime component showed a positive peak around 690 nm and a negative peak around 730 nm, reflecting energy transfer between PSII and PSI. The 100-ps lifetime component showed the largest amplitude, with two broad peaks around 690 nm and 720 nm. Excitation energy was distributed to both PSII and PSI and trapped by P680 and P700 within 100 ps after antenna excitation. The ratio of these two peaks was about 2:3, reflecting the trapping ratio of P680 and P700 in the larger PSI–PSII complex after antenna excitation. According to reduced-minus-oxidized absorption analysis of cytochrome b559 and P700 in the w1 sample, the ratio of PSI to PSII was close to 1:1 in the w1 sample ( Supplementary Table 1 ). These results indicate that PSI accepts a slightly larger amount of excitation energy than PSII in the larger PSI–PSII complex when the PSII reaction center is open. The 570-ps and 2.2-ns components showed a peak at 685 nm, reflecting trapped excitation energy at PSII that was not transferred to PSI. Some PSII might energetically detach from PSI during isolation procedures. The w1 sample showed fast fluorescence decay even in the presence of (3-(3,4-dichlorophenyl)-1,1-dimethylurea) ( Supplementary Fig. 13 ), which indicates that PSII can divert excitation energy to PSI when PSII becomes closed-state in the PSI–PSII complex. The rapid energy migration disappeared when the w1 sample was incubated in 1% α-dodecyl maltoside ( Supplementary Fig. 14 ; Supplementary Note 3 ), indicating detachment of PSII and LHCII from PSI. Figure 3: Fluorescence decay-associated spectra of the w1 sample (20 °C). Decay curves were measured two times with a 2.4-ps interval. Lifetime components were normalized to the lifetime component of the largest amplitude in the sample. Full size image Dynamic response of the PSI–PSII complex to light intensity To elucidate the physiological function of the PSI–PSII complex, we examined the changes in PSI–PSII complexes when the plants were exposed to different light conditions. Intact leaves were corrected under various light conditions, and fluorescence decay-associated spectra were constructed to obtain delayed fluorescence spectra ( Supplementary Figs 15,16 ). After a 14-h dark period, the estimated ratio of PSI–PSII complexes was 46% ( Fig. 4a , dark). When the plants were exposed to growth light (50 μmol photons m −2 s −1 ) for 3 h, the ratio increased to 63% ( Fig. 4a , A). High-light treatment (2,000 μmol photons m −2 s −1 ) resulted in further elevation to 70% ( Fig. 4a , D). These results indicate that an increase in light intensity is accompanied by an increase in PSI–PSII complexes. In contrast, when the light intensity was lowered to 50 μmol photons m −2 s −1 , the ratio of PSI–PSII complexes decreased to 55% within 1 min ( Fig. 4a , E). This indicates that energetic decoupling of PSII from PSI occurs immediately after transfer from high-light to growth-light conditions. Then, the ratio gradually recovered to 62% over 1 h ( Fig. 4a , G), which reflects reformation of PSI–PSII complexes. 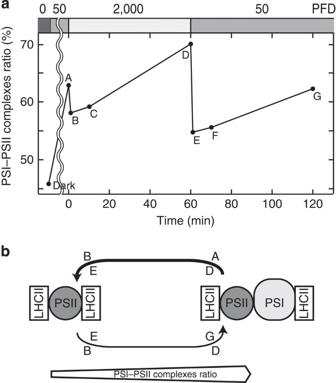Figure 4: Change of the PSI–PSII complexes ratio in the wild-type leaf depending on light conditions. (a) The ratios were determined from the delayed fluorescence spectra and mean lifetimes shown inSupplementary Fig. 15as described inSupplementary Fig. 3and a previous report12. Sample details are shown inSupplementary Fig. 16. Decay curves were measured one time and two times with 1.2-ps interval and 24.4-ps interval, respectively. (b) Schematic representation of the megacomplex formation. The thin arrow represents slow stages such as PSII migration from the grana stack and/or repair processes. The thick arrow represents the fast stage of energetic decoupling of PSII from PSI depending on sudden light changes. Figure 4: Change of the PSI–PSII complexes ratio in the wild-type leaf depending on light conditions. ( a ) The ratios were determined from the delayed fluorescence spectra and mean lifetimes shown in Supplementary Fig. 15 as described in Supplementary Fig. 3 and a previous report [12] . Sample details are shown in Supplementary Fig. 16 . Decay curves were measured one time and two times with 1.2-ps interval and 24.4-ps interval, respectively. ( b ) Schematic representation of the megacomplex formation. The thin arrow represents slow stages such as PSII migration from the grana stack and/or repair processes. The thick arrow represents the fast stage of energetic decoupling of PSII from PSI depending on sudden light changes. Full size image It has been suggested that phosphorylation of LHC and PSII core components is involved in the migration of photosystems between grana stack and stroma thylakoid regions [18] . To investigate the role of phosphorylation of these proteins, we examined the delayed fluorescence of mutants defective in the phosphorylation of individual proteins. Although some perturbations were observed, three mutants ( stn7 , stn8 and tap38 ) related to phosphorylation of the photosystems possessed PSI–PSII complexes ( Supplementary Fig. 17a–c , 6th components) [19] , indicating that phosphorylated LHCII, D1 and D2 are not required for PSI–PSII complex formation. In this study, we elucidated that the PSII-originated delayed fluorescence from PSI is derived from a PSI–PSII complex. Although the molecular structure of the PSI–PSII complex was not clarified in this study, the core antenna of both photosystems might associate directly because mutants deficient in LHCIIs or LHCIs showed the same delayed fluorescence spectra as the wild type. PSII-originated delayed fluorescence from PSI has been observed from various organisms including cyanobacteria and red algae. Our results suggest that PSI–PSII complexes play important roles in a wide range of photosynthetic organisms, not only in red algae [12] , [20] but also in higher plants. We found that excitation energy migrates between PSI and PSII within 100 ps, and that all of the excitation energy at PSII can be potentially transferred to PSI when PSII is closed-state in the complex. This suggests that PSI can quench PSII when PSII is excessively excited. This idea is supported by the observation that PSI–PSII complexes increased under high-light conditions. Quenching of excess energy by PSI might be one of the physiological functions of PSI–PSII complexes. Plant materials The Columbia ecotype of wild-type and mutant A. thaliana were grown at 22 °C under short-day conditions (8 h light, 50 μmol photons m −2 s −1 , white fluorescent lamp) in trays (~5 cm depth) containing layers of horticultural soil (National Federation of Agricultural Cooperative Association, Japan) and expanded vermiculite (Taiheiyo Coal Services and Transportation, Japan). The fertilizer ratio in this mixture was N:P 2 O 5 :K 2 O:MgO=34:135:22:15. Leaves were harvested about 9 weeks after seeding. Mutant seeds were obtained from the Arabidopsis Biological Resource Center. Sample separation using lpCN-PAGE Thylakoid membranes were isolated and solubilized with 1% digitonin (Sigma-Aldrich Japan, Tokyo) at 21 °C as described previously [6] . In brief, leaves were harvested from 80 individual plants. One leaf was used for spectroscopic measurements, and the remaining leaves were used for thylakoid isolation. Leaves were ground in the grinding buffer (50 mM Hepes/KOH pH 7.5, 330 mM sorbitol, 2 mM EDTA, 1 mM MgCl 2 , 5 mM ascorbate, 0.05% bovine serum albumin, 10 mM sodium fluoride) at 4 °C and the homogenate was filtered through Miracloth layers. After centrifugation (5,000 g , 4 min, 4 °C), the pellet was suspended in the shock buffer (50 mM Hepes/KOH pH 7.5, 5 mM sorbitol, 5 mM MgCl 2 , 10 mM sodium fluoride) at 4 °C and the suspension was centrifuged again. The thylakoid pellet was suspended in the storage buffer (50 mM Hepes/KOH pH 7.5, 100 mM sorbitol, 10 mM MgCl 2 , 10 mM sodium fluoride) to a chlorophyll concentration of 1.5 mg ml −1 . The thylakoid membrane was solubilized with 1% digitonin at 0.5 mg chlorophyll per ml in the 25BTH20G buffer (25 mM BisTris/HCl pH 7.0, 20% (w/v) glycerol, 0.25 mg ml −1 Pefabloc SC, 10 mM sodium fluoride) at 21 °C. lpCN-PAGE was performed essentially as described previously [6] . In brief, in separation gel, acrylamide gradient was 3.5–12.5%, where the ratio of bisacrylamide to the total acrylamide was 3%. In stacking gel, total acrylamide concentration was 3%, where the ratio of bisacrylamide to the total acrylamide was 20%. Both gels were prepared using the gel buffer containing 0.5 M 6-aminocaproic acid and 50 mM BisTris/HCl pH 7.0 at 4 °C. Anode buffer contained 50 mM BisTris/HCl pH 7.0 at 4 °C. The only difference from the previous study was that the cathode buffer (50 mM Tricine, 15 mM BisTris/HCl pH 7.0 at 4 °C, 0.05% sodium deoxycholate) did not contain Coomassie Brilliant Blue or dodecyl maltoside because the former acted as a competitive quencher of chlorophyll fluorescence in LHCII, and the latter deteriorated the megacomplex ( Supplementary Fig. 18 ). Note that the stacking gel was polymerized for 40 min above 26 °C. Gel images were captured with a scanner (GT-X970, Epson, Japan), and input levels were adjusted by curve adjustment (Photoshop CS5.1, Adobe Systems, USA). Typically, a black point was set to a default value, and a white point was set to ~200. Intact leaves and bands in lpCN-PAGE were excised and put into quartz tubes of 5-mm diameter under dim-light conditions and stored at −80 °C prior to spectroscopic measurements. Intact leaves for the varying growth light experiment ( Supplementary Fig. 16 ) were excised under each growth light condition and frozen within 10 s. SDS–PAGE and immunoblot analyses were performed as described previously [21] . In brief, the excised lanes of lpCN-PAGE were immersed in a solution containing 1% SDS and 1% 2-mercaptoethanol at 25 °C for 1 h and run on polyacrylamide gels using Laemmli buffer. Total acrylamide concentration was 14%, where the ratio of bisacrylamide to the total acrylamide was 2.6%. The gels were prepared using the gel buffer containing 12.4 mM Tris/HCl pH 6.8 and 0.13% SDS. After electrophoresis, a gel was stained using the silver stain kit (Pierce Silver Stain for Mass Spectrometry, Thermo Scientific, USA) and the remaining gels were used for immunoblot analysis. The proteins were blotted onto polyvinylidene fluoride membranes with transfer buffer (25 mM Tris, 192 mM glycine, 20% methanol). The protein were detected using the Western Lightning Chemiluminescence Reagent Plus (Perkin Elmer, Life Sciences). Antibody dilutions were as follows: PsaA/B (raised against purified PsaA/B [21] , 1:50,000), CP47 (Agrisera AS04 038, 1:3,000), CP43 (Agrisera AS11 1787, 1:3,000), D1 (Agrisera AS01 016, 1:9,000), Lhcb1 (Agrisera AS01 004, 1:5,000), Lhcb2 (Agrisera AS01 003, 1:5,000), Lhcb3 (Agrisera AS01 002, 1:1,000), Lhca3 (Agrisera AS01 007, 1:5,000), Lhca4 (Agrisera AS01 008, 1:5,000), Cyt b 6 (Agrisera AS03 034, 1:15,000). Spectroscopic analyses Time-resolved spectroscopic measurements and analysis were performed as described previously but using a 5-nm optical slit width [22] . The excitation wavelength was 425 nm and the repetition rate was 2.9 MHz, which did not interfere with measurements up to 100 ns (24.4 ps per channel × 4,096 channels). To improve time resolution, time-resolved fluorescence was also measured up to 5 ns (1.2 ps per channel × 4,096 channels) at −196 °C. At 20 °C, time-resolved fluorescence was measured up to 10 ns (2.4 ps per channel × 4,096 channels). The excitation laser intensity was ~0.1 nJ per pulse or less. All experiments were replicated at least two times. Reproducibility of decay curves were verified, and the curves were summed and kinetics were analysed. All samples were measured using the surface-reflection technique ( Supplementary Fig. 19 ) [23] . In brief, fluorescence was corrected at a excitation point on surface of the sample via a narrow slit (0.5 mm width). The excitation and collection position on the sample was adjusted using guide laser and optical stages. In this experimental condition, reabsorption does not affect delayed fluorescence in the PSI wavelength region ( Supplementary Fig. 20 ). On the basis of changes of χ 2 and differences between decay curves and fitting curves [22] , we chose six-component analysis for the −196 °C measurement results, and four-component analysis for the 20 °C measurement results. Final time resolution was about 10 ps. Steady-state fluorescence spectra were measured using an F-2500 spectrophotometer (Hitachi). The optical slit widths for excitation and emission were 10 and 2.5 nm, respectively. For reduced-minus-oxidized absorption measurements [24] , about 3 ml of each excised band from lpCN-PAGE was immersed in the same volume of 25BTH20G buffer [6] with 2% β-dodecyl maltoside for 24 h (4 °C, dark). The extracted solution was dispensed in 1.5-ml aliquots and used for quantitative analysis of cytochrome b559 and P700 in the excised band. Spectra were recorded using a U-3310 spectrophotometer (Hitachi) at room temperature. The optical slit width was 5 nm, and the scan speed was 120 nm min −1 . Hydroquinone and potassium hexacyanoferrate (III) obtained from Nacalai Tesque (Japan) were used as oxidants of cytochrome b559 and P700, respectively. Sodium L -ascorbate was added as a reducing agent. For P700, an extinction coefficient of 64 mM −1 cm −1 was used [25] . For cytochrome b559 , an extinction coefficient of 25 mM −1 cm −1 was used [26] . The chlorophyll concentration and a / b ratio were determined as described previously [27] . In brief, the extracted solution was diluted with 80% acetone, and centrifuged at 18,000 g for 1 min. Absorbance of the supernatant was measured at 646.6 and 663.6 nm and used for calculations. LC–MS/MS analysis For LC–MS/MS analysis, green bands of lpCN-PAGE were cut into slices. The proteins in each gel slice were in-gel digested with trypsin and identified by LC–MS/MS [28] . For the label-free estimate of relative protein abundances in each band from LC–MS/MS data, we used the exponentially modified protein abundance index method [29] . Accession codes : the mass spectrometry proteomics data have been deposited to the ProteomeXchange Consortium [30] via the PRIDE partner repository with the data set identifier PXD001803 . How to cite this article: Yokono, M. et al . A megacomplex composed of both photosystem reaction centres in higher plants. Nat. Commun . 6:6675 doi: 10.1038/ncomms7675 (2015).